Confined molecular catalysts provide an alternative interpretation to the electrochemically reversible demetallation of copper complexes 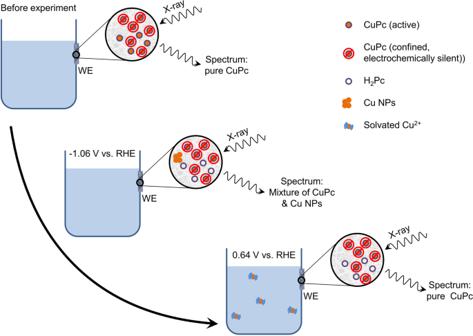Fig. 1: Schematic summary of the alternative interpretation for experimental reported data2. In this scenario, the demetallation ofCuPcis an irreversible process. Likewise, because XAS analysis only probes the Cu element inside the film at the electrode, the normalized spectrum of pureCuPcis recovered after the potential is returned to anodic value, while the Cu atoms constituting the CuNPs have leached from the electrode. Ink preparation Following the reported procedure [2] , 1.6 mg of MWCNTs and 6.4 mg of CuPc (massic ratio CuPc/MW 4:1) were mixed into 2 mL of methanol. In all, 48 μL of Nafion 5% was added and sonicated for 45 min at 20 °C. Film preparation 140 µL of the prepared ink was drop casted on Toray paper (1 cm × 0.5 cm) at room temperature. The electrode was dried in an oven at 100 °C for 30 min. Overall, 0.45 mg of CuPc was deposited on the electrode (0.90 mg/cm 2 ). Electrochemical reduction of CuPc/MWCNT films In an electrochemical cell previously washed with nitric acid, 30 mL of a 0.5 M KHCO 3 solution previously purified (chronopotentiometry at 25 μA cm −2 for 18 h) was added and saturated with 1 atm. CO 2 (pH 7.2). The electrochemical experiment was performed in a three electrodes configuration with CuPc/MWCNT film as the working electrode, a glassy carbon plate as the counter electrode, and a saturated calomel electrode (SCE) was used as the reference electrode. An applied negative potential value of −1.73 V vs. SCE (−1.06 V vs. RHE) was set, with iR compensation, until the current stabilizes. The potential was then set back to −0.03 V vs. SCE (0.64 V vs. RHE) until the current stabilize again. The electrolyte after electrolysis was collected and analyzed by ICP so as to quantify the Cu content and it was compared to an electrolyte prior to the electrochemical experiment (see Supplementary information for details and data analysis).